Bolaform surfactants with polyoxometalate head groups and their assembly into ultra-small monolayer membrane vesicles Surfactants are indispensable in established technologies as detergents or emulsification agents, and also in recent studies for controlling the growth of nanoparticles or for creating nanocarriers. Although the properties of conventional, organic surfactants are thoroughly explored, strong interest persists in surfactants that possess unique features inaccessible for ordinary systems. Here we present dipolar, bolaform surfactants with a head group comprising of 11 tungsten atoms. These novel compounds are characterized by an exceptionally low critical self-organization concentration, which leads to monolayer vesicles with a diameter of only 15 nm, that is, substantially smaller than for any other system. The membrane of the vesicles is impermeable for water-soluble and oil-soluble guests. Control over release kinetics, which can be followed via the quantitative fluorescence quenching of confined fluorophores, is gained by means of pH adjustments. The self-organization of amphiphiles to complex soft-matter structures like micelles, liquid crystals, vesicles or emulsions commands a high degree of research interest, due to its great importance in technology, nanoscience, biology and even medicine. The preparation of novel nanocapsules has received particularly significant attention [1] , [2] , [3] . Systems with so-called monolayer lipid membranes (MLMs) [4] , formed by surfactants bearing two hydrophilic end groups connected by a hydrophobic spacer, also called bolaform amphiphiles (bolas) [5] , [6] , [7] , [8] , have fascinating properties. The survival of archaebacteria under harsh conditions, such as acidic media, anaerobic environments or extreme temperatures, is due to the extraordinary stability of MLMs [9] , [10] . Presently, MLM systems are used with great success for the delivery of ions, drugs or genes and in biosensor devices [4] , [10] , [11] , [12] . As bolas are difficult to isolate from natural sources, there is great interest in their synthesis [9] . It has been shown that synthetic bolas can form many kinds of supramolecular aggregates and that there is a complex relationship between chain composition, spacers and head groups, which crucially influences their self-assembly behavior [4] , [13] , [14] . Single-chained bolas tend to arrange in fibres, ribbons or tubes and doubled-chained bolas form primarily vesicles [13] . Asymmetric bolas with head groups of different sizes tend to arrange selectively in small vesicles with an unsymmetrical monolayer membrane [4] . The development of surfactants containing inorganic entities as multifunctional head groups is an emerging field, which paves the way for novel systems with properties currently not accessible in amphiphile science. Among these, amphiphiles with polyoxometalate (POM) clusters [15] , [16] as head groups show unusual self-assembly behaviour, catalytic activity, interesting magnetic properties and a rich electrochemistry [17] , [18] , [19] , [20] . One further remarkable property of POM surfactants is the exceptional size of the head group and the enhanced electronic contrast between head and chain, which make them suitable as model systems for detailed studies about interfacial self-assembly [21] . Recently, we have reported a double-tailed surfactant comprising the lacunary [PW 11 O 39 ] 3− POM cluster as a head group. In view of the negative charge of the POM head group, [PW 11 O 39 ] 3− , we have set out to prepare a bolaform surfactant with dipolar character by introducing an antipodal, positively charged head group (see Fig. 1 ). 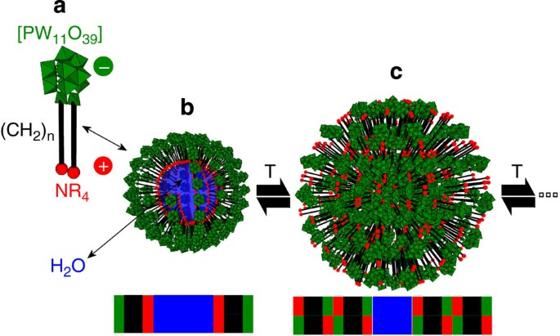Figure 1: Schematic self-assembly behaviour of the POM bolaform surfactant (POMBOLA). (a) The bipolar POMBOLA surfactant reported in this study with an anionic POM head and a cationic ammonium head on opposite ends. (b) MLM vesicles formed by POMBOLA at room temperature. (c) An increase of temperature leads to a structural transformation accompanied by a step-wise growth of the vesicles. Figure 1: Schematic self-assembly behaviour of the POM bolaform surfactant (POMBOLA). ( a ) The bipolar POMBOLA surfactant reported in this study with an anionic POM head and a cationic ammonium head on opposite ends. ( b ) MLM vesicles formed by POMBOLA at room temperature. ( c ) An increase of temperature leads to a structural transformation accompanied by a step-wise growth of the vesicles. Full size image Synthesis of the POMBOLA surfactant A novel POMBOLA surfactant was synthesized in seven steps (see the Methods section and Supplementary Fig. S1 ). In essence, a so-called lacunary POM cluster was reacted with two equivalents of a (CH 2 ) 11 -modified organosilane containing an additional, terminal boc-protected amine group [19] , [22] . Deprotection and protonation using a cation-exchange resin column affords the desired product. The POMBOLA was characterized by nuclear magnetic resonance (NMR) spectroscopy, Fourier transform infrared- and Fourier transform-Raman spectroscopy (see Supplementary Figs S2–7 ). The integrity of the [PW 11 O 39 ] head group is proven by the typical 2:2:1:2:2:2 pattern of its 183 W-NMR signals in combination with the characteristic 31 P-NMR signal at δ =−13.84 ppm. The 1 H-NMR signal at δ =7.57 ppm can be assigned to the terminal NH 3 + groups. It should be noted that the molecular mass of POMBOLA H 3 [PW 11 O 39 (SiC 11 H 22 NH 3 Cl) 2 O] ( M w =3,166.1 g mol −1 ), determined by electron spray ionization mass spectrometry, is much higher than that of conventional, organic bolas. Spontaneous formation of MLM vesicles The concentration dependence of the spontaneous aggregate formation in water was investigated using dynamic light scattering (DLS). At c =8 × 10 −7 mol l −1 , we observe only isolated POMBOLA molecules ( Fig. 2 ) with an average hydrodynamic diameter D H , which fits well to the extension of one single amphiphile chain (~3 nm). Aggregates with D H =16 nm are observed for higher concentrations ( c ≥3 × 10 −6 mol l −1 ) as shown in Fig. 2a . The critical aggregation concentration of POMBOLA is much lower than that of classical ionic surfactants (for example, SDS; 8.3 × 10 −3 mol l −1 ); it even lies below the range of non-ionic, polymeric detergents (for example, Tween 80; 1.2 × 10 −5 mol l −1 ) (ref. 23 ) and represents one of the lowest critical aggregation concentration values known to date [24] . The particle-size distribution remains unchanged and mono-modal up to c =1.1 × 10 −4 mol l −1 (see Supplementary Fig. S8 ). Then, additional, smaller aggregates, eventually micelles, appear ( Fig. 2b ). The nature of the first-formed aggregate was studied in further detail. Transmission electron microscopy (TEM) reveals that the sample consists of spherical objects in the size range of 15–20 nm (see Supplementary Fig. S9 ). A TEM micrograph, recorded at high magnification ( Fig. 2e ), shows that the particles do not have a compact appearance, but rather that of a vesicular structure, as indicated in Figs 1b , 2d . To the best of our knowledge, such small vesicles have not been reported before. The [PW 11 O 39 ] heads of the POMBOLA, which are located at the vesicle surface, give rise to the observation of a very narrow border with unusually high imaging contrast. This hypothesis is strongly supported by line-scan energy-dispersive X-ray (EDX) spectroscopy performed for the W Mα edge ( Fig. 2c , see also Supplementary Fig. S10 ), which shows that the density of tungsten is much higher in the periphery of the vesicles than in the centre. Single vesicles have been resolved for high-resolution TEM measurements on a diluted sample ( Fig. 2f ). 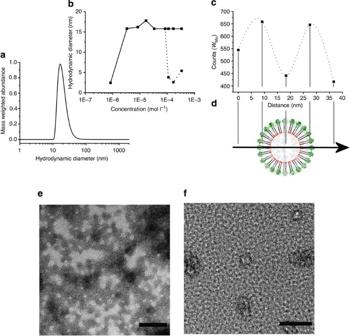Figure 2: MLM vesicle formation. (a) Particle-size distribution curve determined from DLS for the POM bolaform surfactant (POMBOLA) in water atc=8 × 106mol l−1. DLS data are given inSupplementary S2. (b) Aggregate size as a function of amphiphile concentration. (c)WMαline-scan EDX analysis on one single POMBOLA vesicle (d); see alsoSupplementary Fig. S10. (e) TEM micrograph of the POMBOLA vesicles. Scale bar, 100 nm. (f) High-resolution TEM recorded on a diluted sample of vesicles. Scale bar, 50 nm. Figure 2: MLM vesicle formation. ( a ) Particle-size distribution curve determined from DLS for the POM bolaform surfactant (POMBOLA) in water at c =8 × 10 6 mol l −1 . DLS data are given in Supplementary S2 . ( b ) Aggregate size as a function of amphiphile concentration. ( c ) W Mα line-scan EDX analysis on one single POMBOLA vesicle ( d ); see also Supplementary Fig. S10 . ( e ) TEM micrograph of the POMBOLA vesicles. Scale bar, 100 nm. ( f ) High-resolution TEM recorded on a diluted sample of vesicles. Scale bar, 50 nm. Full size image The large electronic contrast of the POM head also facilitates the acquisition of small-angle X-ray scattering (SAXS) from aqueous dispersions using Guinier (ln I vs q 2 ), Porod (log I vs log q ) and Kratky plots ( q 2 I vs q ; data given in Supplementary Figs S11–12 ) (ref. 25 ). As the slope of the Guinier plot is given by− R G 2 /3, one can determine a radius of gyration of R G 8.31 nm for the aggregates described above, in close agreement with the TEM data. As R H is also known (from DLS; see above), we can calculate the ratio ρ = R G / R H , which represents a highly structure-sensitive property reflecting the radial density distribution of the particle [26] . The value of ρ =0.99 thus obtained is very close to that expected for an ideal, hollow sphere with a thin shell ( ρ =1). The ultra-small dimension of the vesicles can be rationalized by the formation of MLMs comprising the giant POM head group together with the primary ammonium groups as the smallest possible hydrophilic head. This combination favors the formation of unsymmetrical membranes with high curvature. If this assumption is correct, one would expect that the outer surface of the vesicular aggregate is characterized by significant negative charge due to the surface-exposed POM clusters ( Fig. 1b ). ζ-Potential measurements confirm this proposition ( Fig. 3a ). As an independent experiment, the metachromatic effect of methylene blue was used as a sensitive probe for the symmetry or asymmetry of MLMs [11] , [27] , [28] . As no blue shift of the absorption band was detected (data given in Supplementary Fig. S13 ), we can conclude that the interior surface of the vesicles is made up of the positive ammonium groups. 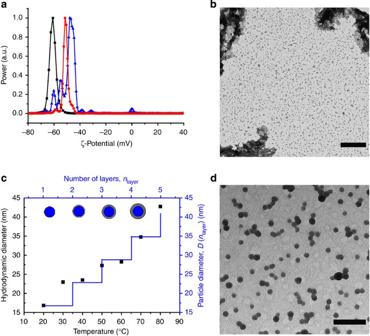Figure 3: Temperature dependence of the self-assembly behaviour. (a) ζ-Potential measurements for three different temperatures: 20 °C (black squares), 50 °C (red circles) and 70 °C (blue triangles). TEM data of aggregates observed at higher temperatures (b, scale bar, 500 nm;d, scale bar, 100 nm). (c) Hydrodynamic diameter as a function of temperature, as determined by DLS (black data points) and as expected for a layer-by-layer growth (blue). Figure 3: Temperature dependence of the self-assembly behaviour. ( a ) ζ-Potential measurements for three different temperatures: 20 °C (black squares), 50 °C (red circles) and 70 °C (blue triangles). TEM data of aggregates observed at higher temperatures ( b , scale bar, 500 nm; d , scale bar, 100 nm). ( c ) Hydrodynamic diameter as a function of temperature, as determined by DLS (black data points) and as expected for a layer-by-layer growth (blue). Full size image Switchable self-assembly behaviour Temperature has a significant and highly unusual influence on the self-organization of our MLM vesicles. DLS measurements indicate that there is a ‘quantized growth’ of the POMBOLA structures for every 15 K in steps of 6 nm, which represents the extension of each POMBOLA unit by an additional surface layer ( Fig. 3d ). This observation is reminiscent of the layer-by-layer method used to produce interesting nanostructures [29] . TEM images reveal that the resulting particles have a more compact character ( Figs 3c , 1c ). The ρ parameter is now 0.72, which is close to the value of 0.775 associated with solid spheres. It should be emphasized that this aggregation process is fully reversible. In addition, we have observed that the particles tend to form large colloidal assemblies due to their uniform size, as shown by TEM micrographs taken at lower magnification ( Fig. 3b ). Host–guest studies Further, unique features of the POMBOLA system were probed by investigating guests brought into the small cavity of the MLM vesicles. The results obtained open new vistas in confinement chemistry, as will be shown below [30] . For example, it is well known that formation of the complex anion [Fe III Fe II (CN) 6 ] − , which is followed by precipitation of Prussian blue, is brought about by mixing solutions of K 4 [Fe II (CN) 6 ] and of Fe III Cl 3 (see Fig. 4a ). If each of these solutions is first entrapped in two separate batches of POMBOLA vesicles, however, and then combined afterwards, no formation of the blue-colored anion [Fe III Fe II (CN) 6 ] − is observed, even after weeks, as documented by visual inspection and spectroscopic measurements ( Fig. 4a ). This experiment shows the exceptional impermeability of the POMBOLA vesicles. The behaviour of entrapped fluorescence probes, like rhodamine 6G (Rh6G), makes the influence of the POMBOLA vesicle confinement evident even by visual inspection ( Fig. 4b ). Although a solution of free Rh6G exhibits the characteristic, strong emission at λ max =550 nm, fluorescence is quenched quantitatively when the dye is located inside the vesicle. We attribute this quenching of the fluorescence to the strong confinement effect and the resulting proximity of the probes to the heavy metal centres contained in the POMBOLA surfactant heads. The same phenomenon is found for other fluorophores like calcein (see Supplementary Fig. S14 ). The emergence of the characteristic fluorescence signal can thus be used as a sensitive tool to decide whether the dye is located inside or outside the vesicle ( Fig. 4c ) and, consequently, to determine release kinetics. The kinetic behaviour is found to depend on the pH value of the aqueous solvent. Under slightly acidic conditions (pH=4.7) vesicles retain their low permeability. At higher pH values, approaching physiological conditions (pH=7.4), however, almost the entire dye is released from the vesicles within minutes. This change can be explained by a partial degradation of the POM group under basic conditions. As evidenced by the behaviour at pH=6, the guest-release rate can be adjusted by using different pH values. 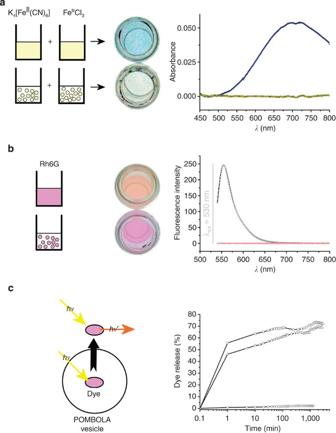Figure 4: Guests confined to the POMBOLA vesicles. (a) [FeIIIFeII(CN)6]−formation experiment using conventional solutions (as reference) and precursors entrapped in POM bolaform surfactant (POMBOLA) vesicles. The characteristic blue colour is not observed when the vesicular solutions are combined. (b) Comparison of a conventional solution of Rh6G to a vesicular solution shows the quantitative quenching of the fluorescence signal. (c) Release kinetics studied at different pH values (circles4.7; triangles6.0; squares7.4), based on the difference in optical properties (fluorescence for free dye, and fluorescence quenching for confined dye). Figure 4: Guests confined to the POMBOLA vesicles. ( a ) [Fe III Fe II (CN) 6 ] − formation experiment using conventional solutions (as reference) and precursors entrapped in POM bolaform surfactant (POMBOLA) vesicles. The characteristic blue colour is not observed when the vesicular solutions are combined. ( b ) Comparison of a conventional solution of Rh6G to a vesicular solution shows the quantitative quenching of the fluorescence signal. ( c ) Release kinetics studied at different pH values (circles 4.7; triangles 6.0; squares 7.4), based on the difference in optical properties (fluorescence for free dye, and fluorescence quenching for confined dye). Full size image The novel POMBOLA surfactant exhibits a unique self-assembly behaviour in water. Monolayer membrane vesicles with low polydispersity have been observed. The spherical vesicles have a diameter of 15 nm making them to the smallest MLM vesicles known to date. The key regarding the formation of aggregates of such small dimensions is the combination of primary ammonium groups as the smallest hydrophilic head group with the giant POM head group. This facilitates the formation of unsymmetrical and highly curved interfaces whereby the POM head groups occupy selectively the outer surface of the MLM membrane ( Fig. 1b ). The vesicular structures show a dynamic self-assembly behaviour as function of temperature resulting in a reversible conversion from MLM vesicles into multilamellar vesicles. Finally, the role of the POMBOLA vesicles as nanocontainers was investigated. It was demonstrated that the membrane of the vesicle is highly impermeable. Hydrophilic, ionic as well as hydrophobic compounds can be encapsulated. The confined, aqueous nanophase leads to interesting confinement effects for encapsulated dye molecules. In the case of fluorescence dyes it was shown that their emission can be quenched quantitatively. The latter phenomenon allowed for a precise differentiation between guest inside or outside the POMBOLA vesicles. Release kinetics triggered by a change in pH value could be observed. Synthesis and materials Starting materials and reagents were purchased from ABCR and Sigma-Aldrich and used without further purification. Tetrahydrofuran was dried over sodium and freshly distilled before use. Dichloromethane was refluxed over CaH 2 and freshly distilled before use. The synthesis route to tert -butyl (11-(triethoxysilyl)undecyl)carbamate 5 is depicted in Supplementary Fig. S1 . Undec-10-en-1-amine 3 and compounds 4 and 5 were synthesized via modified literature methods [31] , [32] , [33] . The purity was confirmed by 1 H NMR spectroscopy. Protection of undec-10-en-1-amine with Boc 2 O ( 4 ) To a solution of 790 mg (4.666 mmol) undec-10-en-1-amine in 10 ml dichloromethane was added 1,020 mg (4.666 mmol) Boc 2 O at 0 °C. Afterwards, a catalytic amount NEt 3 was added. After stirring overnight at room temperature, the solution was evaporated to dryness (1.24 g, 99%). 1 H NMR (CDCl 3 ): δ =5.90–5.70 (m, 1H), 5.05–4.85 (m, 2H), 4.52 (br s, 1H), 3.08 (q, J =6.4, 2H), 2.02 (q, J =7.6, 2H) and 1.50–1.15 (m, 24H). Hydrosilylation of 4 with triethoxysilane ( 5 ) A solution of 1.17 g (4.343 mmol) of compound 4 and 1.21 ml (6.514 mmol) triethoxysilane was degassed with nitrogen for 20 min. Afterwards, five drops of Karstedt’s catalyst were added. After degassing for additional 5 min, the solution was stirred under reflux for 26 h. Evaporation of the solvent and the excess triethoxysilane gave the product, which was used without further purification. 1 H NMR (CDCl 3 ): δ =4.55 (br s, 1H), 3.77 (q, J =6.8, 6H), 3.06 (q, J =6.4, 2H), 1.50–1.10 (m, 36H) and 0.58 (m, 2H). Modification of K 7 [PW 11 O 39 ] with 5 ( 6 ) To a suspension of 2.33 g powdered (Me 4 N) 7 [PW 11 O 39 ] (0.729 mmol) in 800 ml acetonitrile was added 790 mg (1.821 mmol) compound 5 . Then consecutively, 3.64 ml of a 1-M HCl solution was added dropwise. After stirring over night at room temperature, the solution was filtered and the solvent was evaporated. The residue was suspended in water. The precipitate was washed with water, methanol and diethyl ether and dried at air (1.59 g). 1 H NMR (dimethyl sulfoxide (DMSO)-d 6 ): δ =6.71 (t, J =6.0, 2H), 3.11 (s, 36H), 2.88 (q, J =6.4, 24H), 1.60–1.12 (m, 54H), 0.71 (t, J =7.2, 4H). 31 P NMR (DMSO-d 6 ): δ =−13.84. 29 Si NMR (DMSO-d 6 ): δ =−51.20. Synthesis of POMBOLA After dissolving of 530 mg of 6 in acetonitrile the solution was passed through a cation-exchange resin column (Amberlite IR120 H) at a rate of one drop per second. Afterwards, the solution was evaporated to dryness and the product was dried at 80 °C under reduced pressure (470 mg). 1 H NMR (DMSO-d 6 ): δ =7.56 (br s, 6H), 2.77 (sex, J =10.2, 24H), 1.63–1.15 (m, 38H), 0.72 (m, 4H). 31 P NMR (DMSO-d 6 ): δ =−13.84. 29 Si NMR (DMSO-d 6 ): δ =−51.18. 183 W NMR (DMSO-d 6 ): δ =−97.87 (2W), −103.36 (2W), −107.25 (1W), −120.80 (2W), −198.43 (2W), −251.02 (2W). Infrared (attenuated total reflectance, POM region): 1109 (Si-O-Si), 1064 (P-O), 1051 (sh, P-O), 1031 (P-O), 994 (sh, W=O), 982 (sh, W=O), 954 (W=O), 857 (W-O-W), 801 (W-O-W), 771 (W-O-W), 740 (W-O-W), 697 (W-O-W). Electrospray ionization mass spectrometry − : m / z =1546.2 {[PW 11 O 39 (SiC 11 H 22 NH 2 ) 2 O]H} 2− . Elemental analysis (%), observed (calculated for C 22 H 51 N 2 O 40 Si 2 PW 11 ) C, 8.51 (8.54) H, 1.57 (1.66) N, 1.00 (0.91). Instrumentation and methods Characterization techniques The 1 H, 31 P and 29 Si NMR spectra were measured on a Varian Unity Inova 400 spectrometer. The 183 W-NMR spectra were recorded in 10 mm tubes on a Bruker Avance III 600 MHz spectrometer. Raman spectroscopy was performed on a Perkin-Elmer Raman station 400 Raman Spectrometer. Infrared spectra were measured on a Perkin-Elmer Spectrum 100 Fourier transform infrared spectrometer using a Perkin-Elmer Universal attenuated total reflectance sampling accessory. SAXS measurements were conducted with a Bruker AXS Nanostar. The SAXS measurement of the vesicle solution was performed in Mark tubes made of soda lime glass with a diameter of 1 mm. Temperature-dependent measurements were realized with a home-made sample holder. The DLS experiments were performed on a Viscotek 802DLS. The concentration of vesicles was 1 g l −1 . Line-scan EDX data were acquired on a JEOL JEM 2200FS equipped with an EDX detector. TEM images were acquired on a Zeiss Libra 120 at 120 kv acceleration voltage and on a JEOL JEM 2200FS, respectively. Absorption spectroscopy was carried out on a Varian Cary 100. Fluorescence spectra were measured on Varian Carey Eclipse instrument. Confinement studies To a vesicle solution was added an aqueous solution of the hydrophilic molecule (methylene blue, potassium hexacyanoferrate(II), iron(III) chloride, Rh6G and calcein). Afterwards, the solution was sonicated for 20 min with a Bandelin-Sonoplus TT13/F2 ultrasonification device. All solutions have a surfactant concentration of 1 g l −1 and were centrifuged after sonication. The supernatant solutions were used for characterization by DLS, ultraviolet/visible and fluorescence spectroscopy and TEM. How to cite this article: Landsmann, S. et al. Bolaform surfactants with polyoxometalate head groups and their assembly into ultra-small monolayer membrane vesicles. Nat. Commun . 3:1299 doi: 10.1038/ncomms2321 (2012).